Saturated fatty acids regulate retinoic acid signalling and suppress tumorigenesis by targeting fatty acid-binding protein 5 Long chain fatty acids (LCFA) serve as energy sources, components of cell membranes and precursors for signalling molecules. Here we show that these biological compounds also regulate gene expression and that they do so by controlling the transcriptional activities of the retinoic acid (RA)-activated nuclear receptors RAR and PPARβ/δ. The data indicate that these activities of LCFA are mediated by FABP5, which delivers ligands from the cytosol to nuclear PPARβ/δ. Both saturated and unsaturated LCFA (SLCFA, ULCFA) bind to FABP5, thereby displacing RA and diverting it to RAR. However, while SLCFA inhibit, ULCFA activate the FABP5/PPARβ/δ pathway. We show further that, by concomitantly promoting the activation of RAR and inhibiting the activation of PPARβ/δ, SLCFA suppress the oncogenic properties of FABP5-expressing carcinoma cells in cultured cells and in vivo . The observations suggest that compounds that inhibit FABP5 may constitute a new class of drugs for therapy of certain types of cancer. Saturated and unsaturated long chain fatty acids (SLCFA, ULCFA) share common roles as energy sources and key membrane components, but also display distinct biological activities. Hence, while high concentrations of SLCFA trigger acute endoplasmic reticulum stress, induce apoptosis and can lead to insulin resistance and diabetes, ULCFA can protect cells from apoptosis and improve glucose uptake [1] , [2] , [3] , [4] , [5] , [6] , [7] . It was also reported that SLCFA can inhibit, whereas ULCFA can induce proliferation of cancer cells [8] , [9] , [10] , [11] . The molecular mechanisms that underlie distinct activities of different types of LCFA remain poorly understood. In cells, LCFA are associated with fatty acid-binding proteins (FABPs), members of the intracellular lipid-binding proteins (iLBPs) family, which also includes proteins that bind retinol or its transcriptionally active metabolite retinoic acid (RA) [12] , [13] , [14] . Some iLBPs are known to cooperate with specific nuclear receptors. Hence, cellular RA-binding protein 2 (CRABP2) and FABP5, respectively, deliver RA to the two nuclear receptors activated by this hormone: the classical RA receptor RAR and the alternative RA receptor PPARβ/δ (refs 15 , 16 , 17 ). Consequently, RA activates RAR in cells that express a low FABP5/CRABP2 ratio, but is targeted to PPARβ/δ in cells in which this ratio is high [15] , [16] , [17] , [18] , [19] , [20] , [21] . As RAR and PPARβ/δ control different sets of genes, RA can exert distinct and sometimes opposing activities. For example, RA inhibits the growth of carcinoma cells where it functions preferentially through CRABP2 and RAR but promotes proliferation where, due to a high level of FABP5, it activates PPARβ/δ (refs 15 , 16 ). Indeed, FABP5 displays oncogenic activities [22] , [23] , [24] , [25] , [26] , [27] , [28] , [29] . FABP5 is upregulated in multiple types of human cancers [22] , [23] , [24] , [25] as well as in tumours that arise in the MMTV- neu mouse model of breast cancer [30] . In these mice, tumour development is inhibited by genetically decreasing the FABP5/CRABP2 ratio [15] , [16] , [28] . Notably, while FABP5 can bind many lipophilic compounds [15] , [31] , it is mobilized to the nucleus in specific response to PPARβ/δ agonists such as RA and ULCFA, but not on binding of non-PPAR ligands such as SLCFA [15] , [32] , [33] . Here we show that SLCFA and ULCFA differentially regulate the transcriptional activities of RAR and PPARβ/δ, and that FABP5 is a critical mediator of these responses. Both LCFA types displace RA from FABP5 and thereby divert the hormone to RAR and activate this receptor. However, while SLCFA block FABP5 and inhibit PPARβ/δ, ULCFA are delivered by FABP5 to PPARβ/δ to induce its activation. We show further that, by concomitantly activating RAR and inhibiting PPARβ/δ, SLCFA suppress the growth of FABP5-expressing carcinomas. These findings define novel physiological functions for LCFA, provide a rationale for understanding distinct biological activities of SLCFA and ULCFA, and suggest that FABP5 inhibitors may comprise a new class of anticarcinogenic drugs. LCFA regulate transcriptional activation by RAR and PPARβ/δ The activation status of RAR and PPARβ/δ in vivo was examined using mice that globally express β-galactosidase (lacZ) under the control of an RAR response element (RARE–lacZ reporter mice) [34] , and mice that globally express luciferase under the control of a PPAR response element (PPRE–luc reporter mice) [35] . Treatment with RA activated the reporter in multiple tissues of RARE–lacZ mice ( Fig. 1a , Supplementary Fig. 1a ). Co-treatment with RA and with the pan–RAR antagonist AGN193109 attenuated the activation of RAR, verifying the specificity of the response ( Supplementary Fig. 1b ). Examination of responses in PPRE–luc mice revealed that, similarly to the effect of the PPARβ/δ-selective ligand GW1516 (GW), RA upregulated luciferase expression in these mice ( Fig. 1b , Supplementary Fig. 1c ). The data thus demonstrate that RA activates both RAR and PPARβ/δ in vivo . Reporter mice were then crossed with FABP5 −/− mice. Ablation of FABP5 enhanced lacZ expression in RARE reporter mice ( Fig. 1c ), and markedly decreased luciferase expression in PPRE–luc reporters ( Fig. 1d , Supplementary Fig. 1d,e ). As FABP5 does not deliver ligands to other PPAR isotypes [36] , the effect of its ablation in PPRE–luc mice must have specifically stemmed from alterations in the activation of PPARβ/δ. The data thus show that FABP5 suppresses the activation of RAR and promotes the activation of PPARβ/δ in vivo . Importantly, RA failed to upregulate luciferase expression in PPRE–luc mice lacking FABP5 ( Fig. 1d , Supplementary Fig. 1f ), demonstrating that this protein is critical for RA-induced activation of PPARβ/δ. 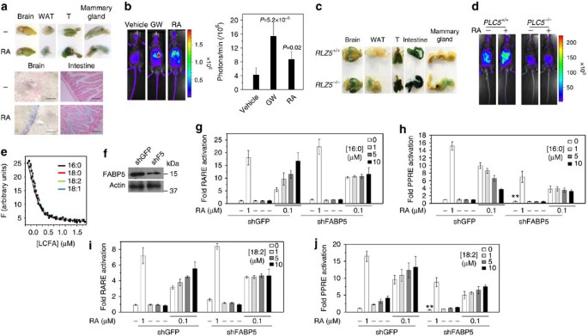Figure 1: LCFAs regulate the transcriptional activity of RAR and PPARβ/δ. (a) X-gal staining of organs (top) and tissue sections (bottom) of RARE–LacZ mice treated with vehicle (−) or RA (1 mg). Representative images out of three mice per group are shown. WAT: white adipose tissue, T: trachea. Magnifications: brain 400 × , intestine 200 × . Scale bars represent 50 μm in brain sections and 100 μm in intestine sections. (b) Left: Images of PPRE–luc mice injected with vehicle, GW1516 (GW), or RA (4 mg). Right: quantitation of data from three mice per group. (c) X-gal staining of organs ofRARE-LacZ+/−/FABP5−/−(RLZ5−/−) andRARE–LacZ+/−/FABP5+/+(RLZ5+/+) mice. Representative images out of six mice per group are shown. (d) Representative images ofPPRE–luc+/−/FABP5−/−(PLC5−/−,n=3) andPPRE–luc+/−/FABP5+/+(PLC5+/+) mice injected with vehicle or RA. (e) Fluorescence competition titrations demonstrating binding of LCFA to FABP5. (f) Immunoblots demonstrating reduced level of FABP5 in HaCaT cells stably expressing FABP5 short hairpin RNA. (g–j) Transactivation assays in HaCaT cells stably expressing shGFP or shFABP5 co-transfected with vectors encoding RARα and RARE-driven luciferase (g,i), or PPARβ/δ and a PPRE-driven luciferase (h,j). Cells were treated with 16:0 (g,h) or 18:2 (i,j) in the presence or absence of RA. Data are mean±s.d. of three independent experiments. **P<0.01 versus non-treated cells, calculated by unpairedt-test. Figure 1: LCFAs regulate the transcriptional activity of RAR and PPARβ/δ. ( a ) X-gal staining of organs (top) and tissue sections (bottom) of RARE–LacZ mice treated with vehicle (−) or RA (1 mg). Representative images out of three mice per group are shown. WAT: white adipose tissue, T: trachea. Magnifications: brain 400 × , intestine 200 × . Scale bars represent 50 μm in brain sections and 100 μm in intestine sections. ( b ) Left: Images of PPRE–luc mice injected with vehicle, GW1516 (GW), or RA (4 mg). Right: quantitation of data from three mice per group. ( c ) X-gal staining of organs of RARE-LacZ +/− /FABP5 −/− ( RLZ5 −/− ) and RARE–LacZ +/− /FABP5 +/+ ( RLZ5 +/+ ) mice. Representative images out of six mice per group are shown. ( d ) Representative images of PPRE–luc +/− /FABP5 −/− ( PLC5 −/− , n =3) and PPRE–luc +/− /FABP5 +/+ ( PLC5 +/+ ) mice injected with vehicle or RA. ( e ) Fluorescence competition titrations demonstrating binding of LCFA to FABP5. ( f ) Immunoblots demonstrating reduced level of FABP5 in HaCaT cells stably expressing FABP5 short hairpin RNA. ( g – j ) Transactivation assays in HaCaT cells stably expressing shGFP or shFABP5 co-transfected with vectors encoding RARα and RARE-driven luciferase ( g , i ), or PPARβ/δ and a PPRE-driven luciferase ( h , j ). Cells were treated with 16:0 ( g , h ) or 18:2 ( i , j ) in the presence or absence of RA. Data are mean±s.d. of three independent experiments. ** P <0.01 versus non-treated cells, calculated by unpaired t -test. Full size image FABP5 can bind multiple ligands, including RA and LCFAs. The equilibrium dissociation constants (Kd) for the association of FABP5 with the SLCFA palmitate (16:0) and stearate (18:0), and the ULCFA linoleate (18:2) and oleate (18:1) were measured by fluorescence competition titrations [37] using bacterially expressed recombinant FABP5 ( Supplementary Fig. 1g ). Binding of the fluorescent lipid 1-anilinonaphthalene-8-sulfonic acid (ANS) to the protein was examined by fluorescence titrations ( Supplementary Fig. 1h ), which yielded a Kd of 70±6.4 nM. The affinities of LCFAs for FABP5 were then assessed by monitoring their ability to displace ANS from the protein ( Fig. 1e ). Kd s for binding of 16:0, 18:0, 18:2, and 18:1 to FABP5 were found to be 20.4±4.2, 15.3±2.4, 19.3±3.3, and 18.5±4.1 nM (data are mean±s.d., n =3), respectively, a somewhat stronger affinity than that of RA (42.3±6.4 nM (ref. 28 )). Human keratinocyte HaCat cells, which express high levels of FABP5 [15] , were used to examine whether FABP5 links cellular responses to its different ligands. Cells were cultured in charcoal-treated medium to deplete them of retinoids and transactivation assays were carried out. Cells were co-transfected either with a vector encoding an RARE-driven luciferase and an expression vector for RARα, or with a PPRE-driven luciferase and an expression vector for PPARβ/δ, treated with LCFA, and luciferase activity was measured. In the absence of RA, neither SLCFA nor ULCFA affected the activity of RAR ( Fig. 1g,i ). SLCFA also did not activate PPARβ/δ ( Fig. 1h ) but, as previously reported [32] , [38] , ULCFAs functioned as agonists for this receptor ( Fig. 1j , Supplementary Fig. 1i ). Strikingly, in the presence of RA, treatment with <10 μM concentrations of all LCFAs modulated the transcriptional activities of both receptors. Both SLCFA- and ULCFA-activated RAR ( Fig. 1g,i ). PPARβ/δ was inhibited by SLCFA ( Fig. 1h ) but activated by ULCFA ( Fig. 1j ). A HaCaT cell line in which the expression of FABP5 is stably decreased was then generated ( Fig. 1f ). Lowering the level of FABP5 abrogated the ability of both 16:0 and 18:2 to activate RAR in the presence of RA ( Fig. 1g,i ). Reducing FABP5 expression decreased the activity of PPARβ/δ even in the absence of RA, indicating that cells contain other endogenous PPARβ/δ ligands that rely on FABP5 for their nuclear delivery ( Fig. 1h,j ). Decreasing the expression of FABP5 also diminished the ability of both SLCFA and ULCFA to regulate RA-dependent PPARβ/δ activity ( Fig. 1h,j ). Modulation of the transcriptional activities of RAR and PPARβ/δ by LCFA was further examined by monitoring their effects on expression of endogenous target genes for these receptors in NaF mammary carcinoma cells. NaF cells are derived from tumours that arise in the MMTV– neu mouse model of breast cancer [30] and they express a high level of FABP5 (ref. 16 ). Similarly to their effects in transcriptional activation assays, both SLCFA and ULCFA induced the expression of the RAR target genes Rarb and Cyp26a ( Fig. 2a,b , and Supplementary Fig. 2a–c ). Also in accordance with transactivation assays, SLCFA decreased ( Fig. 2c , and Supplementary Fig. 2a,b ), and ULCFA increased ( Fig. 2d , Supplementary Fig. 2c ) the expression of PPARβ/δ target genes Pdpk1 and Pln2 . Cells were then treated with Triacsin C (TriC), an inhibitor of fatty acyl CoA ligase, the enzyme that catalyses the first step in fatty acid metabolism [39] . TriC elevated the level of total free fatty acids in the cells by about twofold ( Supplementary Fig. 2d ) and augmented the respective activities of both SLCFA and ULCFA ( Fig. 2e–h , and Supplementary Fig. 2e,f ). The data thus demonstrate that these effects are exerted by the LCFAs themselves and not by their metabolic products. Notably, TriC upregulated the expression of RAR target genes even in the absence of ectopic administration of LCFA ( Fig. 2e,f ), indicating that RA signalling is controlled by alterations in endogenous LCFA levels. TriC treatment per se did not significantly affect the expression of PPARβ/δ targets ( Fig. 2g,h ), likely reflecting that TriC elevates the levels of both SLCFA, which inhibit, and ULCFA, which activate PPARβ/δ, resulting in an overall neutral effect. 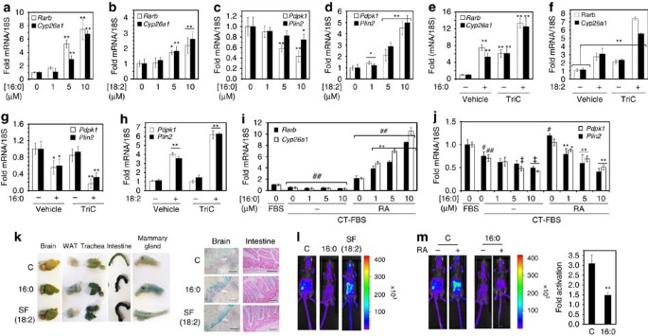Figure 2: Dietary LCFA regulate the transcriptional activity of RAR and PPARβ/δ. (a–d) Levels of mRNA of RAR target genes (a,b) and PPARβ/δ target genes (c,d) in NaF cells treated with 16:0 (a,c) or 18:2 (b,d) for 6 h. (e–h) mRNA for RAR targets (e,f) and PPARβ/δ targets (g,h) in NaF cells treated with vehicle, 16:0 (10 μM;e,g) or 18:2 (10 μM;f,h) for 6 h in the absence or presence of Triacsin C (TriC, 5 μM). Data in (a–h) are mean±s.d. (n=3). *P<0.05, **P<0.01 versus untreated controls. (i,j) mRNA for RAR targets (i) or PPARβ/δ targets (j) in NaF cells cultured in media supplemented with 10% FBS or 10% FBS depleted of retinoids (CT-FBS) treated with 16:0 in the absence or presence of RA (0.2 μM). Mean±s.d. (n=3). #P<0.05, ##P<0.01 versus FBS. *P<0.05, **P<0.01 versus cells cultured in CT-FBS+RA.P<0.01 versus CT-FBS. (k) representative images (out ofn=6) demonstrating X-gal stained organs (left) and tissue sections (right) harvested from RAR-LacZ mice fed control chow (C), 16:0- or SF/18:2-enriched diets for a week. Scale bars represent 50 μm in brain sections and 100 μm in intestine sections. (l) Representative images (out ofn=6) of PPRE-luc mice fed different diets for a week. (m) Left: Mice fed chow or 16:0-enriched diet for a week were injected with RA and imaged 6 h later (left). Right: fold activation. Mean±s.e.m. (n=6).P-values in all panels were calculated using unpairedt-test. Figure 2: Dietary LCFA regulate the transcriptional activity of RAR and PPARβ/δ. ( a – d ) Levels of mRNA of RAR target genes ( a , b ) and PPARβ/δ target genes ( c , d ) in NaF cells treated with 16:0 ( a , c ) or 18:2 ( b , d ) for 6 h. ( e – h ) mRNA for RAR targets ( e , f ) and PPARβ/δ targets ( g , h ) in NaF cells treated with vehicle, 16:0 (10 μM; e , g ) or 18:2 (10 μM; f , h ) for 6 h in the absence or presence of Triacsin C (TriC, 5 μM). Data in ( a – h ) are mean±s.d. ( n =3). * P <0.05, ** P <0.01 versus untreated controls. ( i , j ) mRNA for RAR targets ( i ) or PPARβ/δ targets ( j ) in NaF cells cultured in media supplemented with 10% FBS or 10% FBS depleted of retinoids (CT-FBS) treated with 16:0 in the absence or presence of RA (0.2 μM). Mean±s.d. ( n =3). # P <0.05, ## P <0.01 versus FBS. * P <0.05, ** P <0.01 versus cells cultured in CT-FBS+RA. P <0.01 versus CT-FBS. ( k ) representative images (out of n =6) demonstrating X-gal stained organs (left) and tissue sections (right) harvested from RAR-LacZ mice fed control chow (C), 16:0- or SF/18:2-enriched diets for a week. Scale bars represent 50 μm in brain sections and 100 μm in intestine sections. ( l ) Representative images (out of n =6) of PPRE-luc mice fed different diets for a week. ( m ) Left: Mice fed chow or 16:0-enriched diet for a week were injected with RA and imaged 6 h later (left). Right: fold activation. Mean±s.e.m. ( n =6). P -values in all panels were calculated using unpaired t -test. Full size image FABP5 and RA are critical for LCFA function NaF cells express FABP3 and FABP5 but the latter displays a markedly higher level ( Supplementary Fig. 2g ). Decreasing FABP5 expression in NaF cells ( Supplementary Fig. 2h ) upregulated the RAR target gene Rarb ( Supplementary Fig. 2i ), and suppressed the PPARβ/δ target gene Pdpk1 ( Supplementary Fig. 2j ). The pan–RAR antagonist LE540 abolished the ability of 16:0 to induce RAR targets ( Supplementary Fig. 3a ) but had no effect on the responsiveness of PPARβ/δ target genes ( Supplementary Fig. 3b ). These data demonstrate that induction of RAR target genes by LCFA does not stem from an RAR-independent function of these compounds. These observations also show that RAR is not involved in the modulation of PPARβ/δ activity by 16:0. To examine whether RA is necessary for these effects, cells were depleted of retinoids by culturing in charcoal-treated medium. The depletion decreased the expression of both RAR and PPARβ/δ target genes ( Fig. 2i,j ). 16:0 did not induce the expression of RAR target genes in the absence of retinoids, and the response was restored following replenishment with RA ( Fig. 2i ). Unlike the absolute RA dependence of the responsiveness of RAR targets, 16:0 downregulated the expression of PPARβ/δ targets even in the absence of retinoids ( Fig. 2j ). These observations likely reflect that, in contrast with CRABP2 and RAR, which are specifically activated by RA, FABP5 and PPARβ/δ can be activated by other endogenous ligands. Hence, 16:0 displaces all PPARβ/δ ligands from FABP5. RARE–lacZ and PPRE–luc reporter mice were separated into three groups, which were fed a regular chow, a diet enriched in 16:0, or a diet enriched with safflower oil in which the predominant fatty acid is 18:2 (SF/18:2). Feeding RARE–lacZ mice with diets enriched with either 16:0 or SF/18:2 markedly enhanced X-gal staining, demonstrating the activation of RAR ( Fig. 2k , Supplementary Fig. 4a ). In PPRE–luc reporter mice, 16:0-enriched diet decreased, and SF/18:2-enriched diet increased PPAR activation ( Fig. 2l , Supplementary Fig. 4b ). Strikingly, PPRE–luc mice fed 16:0-enriched diet displayed a markedly reduced response to RA-induced PPAR activation ( Fig. 2m , Supplementary Fig. 4c ). Hence, dietary SLCFA and ULCFA differentially regulate RA signalling in vivo . LCFA differentially modulate cancer cell growth Considering the pro-proliferative activities of the FABP5/PPARβ/δ path [27] , [28] , [29] , the opposing effects of SLCFA and ULCFAs on PPARβ/δ activation suggest that they may differentially modulate cell growth. Indeed, SLCFA suppressed, while ULCFA facilitated NaF cell proliferation ( Fig. 3a,b ). Normal human mammary epithelial cells (HMEC) and MCF-7 mammary carcinoma cells, which express low levels of FABP5, NaF and MBA-MD-231 (231) mammary carcinoma cells and PC3M prostate cancer cells, which highly express the binding protein ( Fig. 3c ) were used to examine the involvement of FABP5 in these opposing effects of the two types of LCFA. 16:0 downregulated the expression of the RAR target gene Rarb and upregulated the PPARβ/δ target Pdpk1 in PC3M and 231 cells but not in MCF-7 cells ( Fig. 3d ). RA facilitated proliferation of 231 and PC3M cells, but not of HMEC and MCF-7 cells ( Fig. 3e ). Strikingly, SLCFA potently inhibited the growth of 231 and PC3M cells, but had no effect on proliferation of either HMEC or MCF-7 ( Fig. 3f , Supplementary Fig. 5a ). This activity was abolished on depletion of retinoids and restored on replenishing depleted media with RA ( Fig. 3g ). 18:2 promoted the growth of the FABP5-expressing 231 and PC3M cells but, similarly to SLCFA, had no effect on growth of MCF-7 and HMEC cells ( Fig. 3h ). Both RA and 18:2 promoted cell proliferation when administered alone, and the activity was additive when these two PPARβ/δ ligands were added together ( Fig. 3i ). Treatment of cells with the PPARβ/δ antagonist, PT-S58 (ref. 40 ), inhibited cell proliferation with an additive effect observed on co-treatment with LCFA ( Fig. 3j,k ). Moreover, despite the inhibition of PPARβ/δ in the presence of PT-S58, 18:2 suppressed cell proliferation ( Fig. 3k ). Considering that PT-S58 inhibits PPARβ/δ (ref. 40 ) but does not associate with FABP5, the activities of LCFA in the presence of the inhibitor likely stemmed from the activation of RAR. Taken together, the data indicate that, by binding to FABP5, both SLCFA and ULCFA activate RAR by shifting RA towards this nuclear receptor. 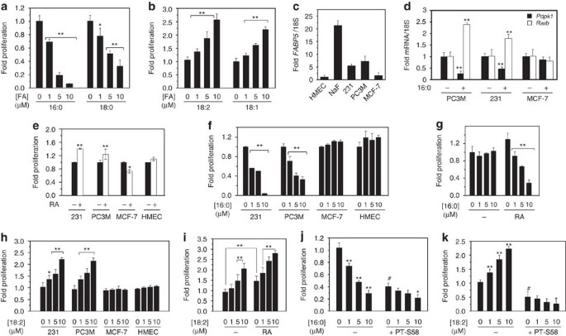Figure 3: SLCFA inhibit and ULCFA induce carcinoma cell growth. (a,b) NaF cells were treated with 16:0, 18:0, 18:2, or 18:1 for 4 days. Proliferation was assessed by MTT assays. (c) FABP5 mRNA in normal human mammary epithelial cells (HMEC), NaF, MDA-MB-231 and MCF-7 mammary carcinoma cells, and PC3M prostate carcinoma cells. (d)Pdpk1andRarbmRNA in denoted cells treated with 16:0 (10 μM, 6 h). (e) Cells were treated with vehicle (−) or RA (1 μM) for 4 days and proliferation assessed by MTT assays. (f) Effect of 16:0 (4 days) on proliferation of denoted cells. (g) Cells were cultured in CT-FBS, treated with 16:0 in the absence or presence of RA (0.2 μM, 4 days), and proliferation assessed by MTT assays. **P<0.01, by unpairedt-test versus cells cultured in CT-FBS replenished with RA. (h) Effect of 18:2 (4 days) on proliferation of denoted cells assessed by MTT assays. (i) Cells were cultured in CT-FBS, co-treated with 18:2 and RA (0.2 μM) for 4 days and proliferation assessed by MTT assays. (j,k) Effect of 16:0 (j) or 18:2 (k) on proliferation of NaF cell in the presence or absence of the PPARβ/δ antagonist PT-S58 (5 μM). #P<0.01 versus untreated control, *P<0.05 versus PT-S58 treatment without LCFA. Data in all panels are Mean±s.d. *P<0.05, **P<0.01 versus the respective control.P-values were calculated by unpairedt-test. Figure 3: SLCFA inhibit and ULCFA induce carcinoma cell growth. ( a , b ) NaF cells were treated with 16:0, 18:0, 18:2, or 18:1 for 4 days. Proliferation was assessed by MTT assays. ( c ) FABP5 mRNA in normal human mammary epithelial cells (HMEC), NaF, MDA-MB-231 and MCF-7 mammary carcinoma cells, and PC3M prostate carcinoma cells. ( d ) Pdpk1 and Rarb mRNA in denoted cells treated with 16:0 (10 μM, 6 h). ( e ) Cells were treated with vehicle (−) or RA (1 μM) for 4 days and proliferation assessed by MTT assays. ( f ) Effect of 16:0 (4 days) on proliferation of denoted cells. ( g ) Cells were cultured in CT-FBS, treated with 16:0 in the absence or presence of RA (0.2 μM, 4 days), and proliferation assessed by MTT assays. ** P <0.01, by unpaired t -test versus cells cultured in CT-FBS replenished with RA. ( h ) Effect of 18:2 (4 days) on proliferation of denoted cells assessed by MTT assays. ( i ) Cells were cultured in CT-FBS, co-treated with 18:2 and RA (0.2 μM) for 4 days and proliferation assessed by MTT assays. ( j , k ) Effect of 16:0 ( j ) or 18:2 ( k ) on proliferation of NaF cell in the presence or absence of the PPARβ/δ antagonist PT-S58 (5 μM). # P <0.01 versus untreated control, * P <0.05 versus PT-S58 treatment without LCFA. Data in all panels are Mean±s.d. * P <0.05, ** P <0.01 versus the respective control. P -values were calculated by unpaired t -test. Full size image In accordance with the pronounced pro-carcinogenic activities of FABP5 (refs 15 , 28 ), decreasing the expression of the protein in NaF cells ( Supplementary Fig. 2h ) inhibited proliferation ( Fig. 4a , Supplementary Fig. 5b ), converted RA from a pro- to an anti-proliferative agent ( Fig. 4b ), hampered formation of colonies in soft agar ( Fig. 4c , Supplementary Fig. 5c ) and suppressed tumour development in a xenograft mouse model ( Fig. 4d ). Treatment of NaF cells with 16:0 inhibited their growth ( Fig. 4e , Supplementary Fig. 5b ), triggered apoptosis ( Fig. 4f,g ) and markedly suppressed colony formation ( Fig. 4h ). These anti-oncogenic activities of 16:0 were markedly diminished in cells in which FABP5 expression was decreased ( Fig. 4e–g , Supplementary Fig. 5b ). Ectopic expression of FABP5 in MCF-7 cells induced cell proliferation ( Fig. 4i ) and suppressed apoptosis ( Fig. 4j ). Strikingly, unlike parental MCF-7 cells, overexpression of FABP5 rendered these cells sensitive to 16:0-induced growth arrest and apoptosis ( Fig. 4i,j , Supplementary Fig. 5d ). Ectopic expression of another FABP, FABP4 ( Supplementary Fig. 5e ), did not compensate for loss of FABP5 ( Supplementary Fig. 5f ), indicating that FABP5 is a specific mediator of the growth-inhibitory activity of 16:0. 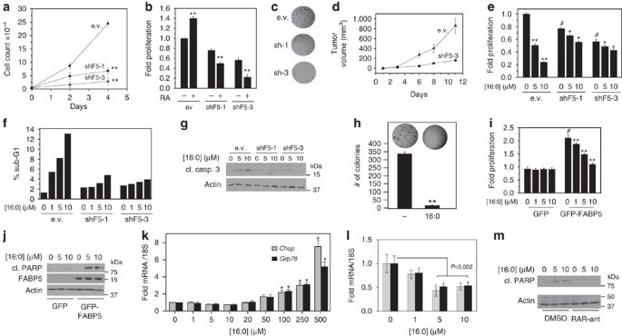Figure 4: FABP5 mediates SLCFA-induced growth arrest and apoptosis. (a) Proliferation of cells expressing varying levels of FABP5 was assessed by cell counting. Mean±s.d. (n=4). **P<0.01, by unpairedt-test versus e.v. expressing cells. (b) MTT assays in cells treated with vehicle or RA (1 μM, 4 days). Mean±s.d. (n=4). **P<0.01, by unpairedt-test versus untreated cells. (c) Representative image (out of 3) of colonies formed in soft agar by NaF lines with varying expression levels of FABP5. SeeSupplementary Fig. S5bfor colony counts. (d) NaF cells (2 × 106) stably expressing empty vector or vector encoding FABP5 short hairpin RNA (shF5-3,Supplementary Fig. S2h) were transplanted into the mammary fat pad of NCr athymic female mice (n=5). Tumour growth was monitored. Mean ±s.e.m. (e) MTT assays in NaF cells treated with 16:0 (4 days). Mean±s.d. (n=4). *P<0.05, **P<0.01 versus untreated control, #P<0.01 versus e.v. control.P-values were calculated by unpairedt-test. (f) Cells were treated with 16:0 for 4 days and apoptosis evaluated by FACS analyses. Data from one out of four experiments are shown. (g) Immunoblots of cleaved caspase 3 in NaF lines treated with 16:0 for 4 days. (h) Representative image (out of 3) of colonies formed in soft agar by NaF cells treated with vehicle (−) or 16:0 (10 μM). **P<0.01 by unpairedt-test. (i) MTT assays in MCF-7 cells overexpressing GFP-FABP5 or GFP control and treated with 16:0 (8 days). Mean±s.d. (n=4). *P<0.05, **P<0.01 versus untreated control, #P<0.01 versus empty vector (e.v.) control. (j) Immunoblots of cleaved PARP in MCF-7 cells overexpressing GFP-FABP5 or GFP control and treated with 16:0 for 8 days. (k) Levels ofChopandGrp78mRNA in NaF cells treated with varying concentrations of 16:0 for 8 h. Mean ±s.d. (n=3). *P<0.05, *P<0.01 by unpairedt-test. (l) Levels ofChopandGrp78mRNA in NaF cells treated with 16:0 for 4 days. (m) Immunoblots of cleaved PARP in NaF cells treated with 16:0 for 4 days in the presence or absence of antagonists for RARα (BMS19614), RARβ (LE 135), or RARγ (MM 11253) (1 μM each). Immunoblots in panels (g,j,m) are representative of 3 independent experiments. Figure 4: FABP5 mediates SLCFA-induced growth arrest and apoptosis. ( a ) Proliferation of cells expressing varying levels of FABP5 was assessed by cell counting. Mean±s.d. ( n =4). ** P <0.01, by unpaired t -test versus e.v. expressing cells. ( b ) MTT assays in cells treated with vehicle or RA (1 μM, 4 days). Mean±s.d. ( n =4). ** P <0.01, by unpaired t -test versus untreated cells. ( c ) Representative image (out of 3) of colonies formed in soft agar by NaF lines with varying expression levels of FABP5. See Supplementary Fig. S5b for colony counts. ( d ) NaF cells (2 × 10 6 ) stably expressing empty vector or vector encoding FABP5 short hairpin RNA (shF5-3, Supplementary Fig. S2h ) were transplanted into the mammary fat pad of NCr athymic female mice ( n =5). Tumour growth was monitored. Mean ±s.e.m. ( e ) MTT assays in NaF cells treated with 16:0 (4 days). Mean±s.d. ( n =4). * P <0.05, ** P <0.01 versus untreated control, # P <0.01 versus e.v. control. P -values were calculated by unpaired t -test. ( f ) Cells were treated with 16:0 for 4 days and apoptosis evaluated by FACS analyses. Data from one out of four experiments are shown. ( g ) Immunoblots of cleaved caspase 3 in NaF lines treated with 16:0 for 4 days. ( h ) Representative image (out of 3) of colonies formed in soft agar by NaF cells treated with vehicle (−) or 16:0 (10 μM). ** P <0.01 by unpaired t -test. ( i ) MTT assays in MCF-7 cells overexpressing GFP-FABP5 or GFP control and treated with 16:0 (8 days). Mean±s.d. ( n =4). * P <0.05, ** P <0.01 versus untreated control, # P <0.01 versus empty vector (e.v.) control. ( j ) Immunoblots of cleaved PARP in MCF-7 cells overexpressing GFP-FABP5 or GFP control and treated with 16:0 for 8 days. ( k ) Levels of Chop and Grp78 mRNA in NaF cells treated with varying concentrations of 16:0 for 8 h. Mean ±s.d. ( n =3). * P <0.05, * P <0.01 by unpaired t -test. ( l ) Levels of Chop and Grp78 mRNA in NaF cells treated with 16:0 for 4 days. ( m ) Immunoblots of cleaved PARP in NaF cells treated with 16:0 for 4 days in the presence or absence of antagonists for RARα (BMS19614), RARβ (LE 135), or RARγ (MM 11253) (1 μM each). Immunoblots in panels ( g , j , m ) are representative of 3 independent experiments. Full size image It is well established that, at high concentrations, SLCFA induce apoptosis by triggering endoplasmic reticulum stress [1] , [2] , [6] . Indeed, an 8 h treatment with >50 μM 16:0 increased the expression of the endoplasmic reticulum stress markers Chop and Grp78 ( Fig. 4k ). However, while 16:0-induced apoptosis at <10 μM ( Fig. 4f,g ), it did not trigger endoplasmic reticulum stress at these concentrations. In fact, treatment with low concentrations of 16:0 reduced the expression levels of both Chop and Grp78 ( Fig. 4l ). Induction of apoptosis in NaF cells and in MCF-7 cells ectopically expressing FABP5, in response to ≤10 μM concentrations of 16:0 was abolished in the presence of antagonists of RARα, β or γ ( Fig. 4m , Supplementary Fig. 5d ). Hence, at low levels, 16:0 induces apoptosis through controlling RA signalling and not via induction of endoplasmic reticulum stress. 16:0 induces genome-wide regulation of cancer-related genes NaF cells, cultured in delipidated medium, were treated with the PPARβ/δ-selective agonist GW1516 (GW), the pan–RAR agonist 4-[(E)-2-(5,5,8,8-tetramethyl-6,7-dihydronaphthalen-2-yl)prop-1-enyl]benzoic acid (TTNPB) or RA (4 h., 1 μM each). Transcriptome analyses (Affymetrix Mouse Gene 2.1 ST Arrays) revealed that 1,047 and 1,474 genes were commonly regulated by RA and GW1516 and RA and TTNPB, respectively ( Supplementary Fig. 6a ). Notably, more genes were regulated by RA (3,960 genes) than by either GW (1,979 genes) or TTNPB (2,598 genes). Transcriptome analyses were also carried out in cells treated with 16:0 (10 μM, 4 h) in the presence of retinoids. The analysis identified 258 and 446 genes commonly regulated by 16:0 and GW1516 and 16:0 and TTNPB, respectively ( Fig. 5a,b ). Hierarchical clustering identified 69 genes whose expression was upregulated by GW1516 and downregulated by 16:0 ( Fig. 5c , Supplementary Data 1 ), and 51 genes that were upregulated by both TTNPB and 16:0 ( Fig. 5d , Supplementary Data 2 ). The data thus show that the expression of a substantial cohort of PPARβ/δ target genes is negatively regulated by 16:0 while many RAR target genes are induced by this LCFA. Strikingly, expression of all 120 genes regulated by 16:0 and GW1516 and by 16:0 and TTNPB were upregulated by RA ( Fig. 5e , Supplementary Data 1 , and Supplementary Data 2 ). 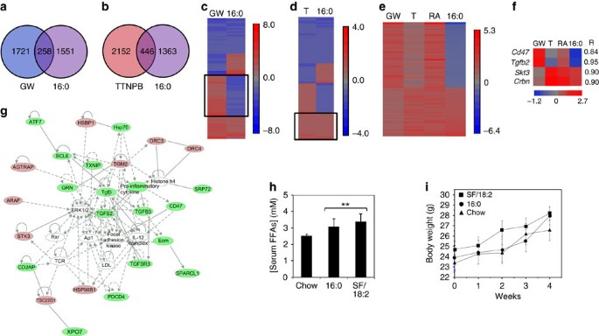Figure 5: 16:0-regulated cancer-related PPARβ/δ and RAR target genes. (a–g) NaF cells were treated with GW1516 (GW; 1 μM), 16:0 (10 μM)., RA (1 μM), or TTNPB (T; 1 μM) for 4 h. Changes in gene expression were analysed using Affymetrix Mouse Gene 2.1 ST Arrays (Affymetrix, USA). (a) Venn diagram showing genes co-regulated by GW and 16:0. (b) Venn diagram showing overlap of genes regulated by TTNPB (T) and 16:0. (c) Hierarchical clustering of genes regulated by GW and 16:0. Boxed: genes upregulaed by GW and downregulated by 16:0. (d) Hierarchical clustering of genes regulated by TTNPB and 16:0. Boxed: genes upregulaed by both TTNPB and 16:0. (e) Heatmap representing expression of genes boxed in c and d regulated by 16:0, TTNPB, GW and RA. (f) Validation of microarray data. Heatmap showing mRNA levels of denoted genes, measured by qPCR. Data is presented as log2 of the 2−ΔΔCTratio and the correlation (R) to the array signal intensity is indicated. Mean±s.d. (n=4). (g) Predicted network of genes with known function in cellular development, cancer and embryonic development (P=2.2 × 10−4) affected by 16:0 treatment in NaF cells. Arrows indicate activation. Lines ending in short perpendicular lines indicate repression. Red shapes and green shapes indicate upregulated and downregulated genes, respectively. Solid and dashed lines indicate direct and indirect interactions, respectively. (h) Concentrations of free FAs in serum of mice fed chow or diets enriched with 16:0 or SF/18:2 for 4 weeks. Mean±s.e.m. (n=6).**P<0.01 calculated by unpairedt-test. (i) Body weights of mice fed denoted diets. Mean±s.e.m. (n=6). Figure 5: 16:0-regulated cancer-related PPARβ/δ and RAR target genes. ( a – g ) NaF cells were treated with GW1516 (GW; 1 μM), 16:0 (10 μM)., RA (1 μM), or TTNPB (T; 1 μM) for 4 h. Changes in gene expression were analysed using Affymetrix Mouse Gene 2.1 ST Arrays (Affymetrix, USA). ( a ) Venn diagram showing genes co-regulated by GW and 16:0. ( b ) Venn diagram showing overlap of genes regulated by TTNPB (T) and 16:0. ( c ) Hierarchical clustering of genes regulated by GW and 16:0. Boxed: genes upregulaed by GW and downregulated by 16:0. ( d ) Hierarchical clustering of genes regulated by TTNPB and 16:0. Boxed: genes upregulaed by both TTNPB and 16:0. ( e ) Heatmap representing expression of genes boxed in c and d regulated by 16:0, TTNPB, GW and RA. ( f ) Validation of microarray data. Heatmap showing mRNA levels of denoted genes, measured by qPCR. Data is presented as log2 of the 2 −ΔΔCT ratio and the correlation (R) to the array signal intensity is indicated. Mean±s.d. ( n =4). ( g ) Predicted network of genes with known function in cellular development, cancer and embryonic development ( P =2.2 × 10 −4 ) affected by 16:0 treatment in NaF cells. Arrows indicate activation. Lines ending in short perpendicular lines indicate repression. Red shapes and green shapes indicate upregulated and downregulated genes, respectively. Solid and dashed lines indicate direct and indirect interactions, respectively. ( h ) Concentrations of free FAs in serum of mice fed chow or diets enriched with 16:0 or SF/18:2 for 4 weeks. Mean±s.e.m. ( n =6). ** P <0.01 calculated by unpaired t -test. ( i ) Body weights of mice fed denoted diets. Mean±s.e.m. ( n =6). Full size image Validating the transcriptome analysis, quantitative real-time PCR showed that the PPARβ/δ target genes Cd47 and Tgfb2 were downregulated, and expression of the RAR target genes Skt3 and Cereblon ( Crbn ) increased on treatment with 16:0 ( Fig. 4f ). Functional analyses of the 120 genes regulated by 16:0 in common with GW1516 and TTNPB (Ingenuity Pathway Analysis) indicated that the most significantly enriched network is ‘cellular development, cancer and embryonic development’ ( P =0.0002). Notably, most genes in this network were downregulated by 16:0 treatment ( Fig. 5g , green), implying an anti-oncogenic activity. 16:0 suppresses tumor growth in vivo Female NCr athymic mice were separated into three groups and fed a regular chow diet, a diet enriched with 16:0, or a SF/18:2-enriched diet. Following a week of feeding, NaF cells were injected into the mammary fat pad and tumor growth was monitored. Consumption of either LCFA-enriched diet elevated serum levels of free fatty acids ( Fig. 5h ). Mice in the three groups consumed similar amounts of food ( Supplementary Fig. 6b ), and displayed similar weight gain ( Fig. 5i ). Total FFA levels in tumours that arose in mice fed either of the LCFA-enriched diets were similarly elevated ( Supplementary Fig. 6c ), but the level of 16:0 was higher only in tumours of mice fed 16:0-enriched diet ( Fig. 6a ). Strikingly, tumour development was markedly suppressed in mice fed 16:0-enriched diet versus in mice fed either regular chow or SF/18:2-enriched diet ( Fig. 6b ). While not statistically significant, tumour development appeared to be facilitated in mice fed SF/18:2-enriched diet. In line with their opposing effects on the activity of PPARβ/δ in cultured cells, tumours that arose in mice fed 16:0-enriched and SF/18:2-enriched diets, respectively, expressed higher and lower levels of the pro-proliferative PPARβ/δ target genes Pdpk1 , Vegfa, Tgfb2 and Cd47 as compared with tumours in chow-fed animals ( Fig. 6c,e ). Tumours in mice fed either 16:0 or SF/18:2 expressed higher levels of the RAR target genes Rarb , Caspase 9 , Skt3 and Crbn , although the effect of 16:0 was more pronounced than that of SF/18:2 ( Fig. 6d,e , Supplementary Fig. 6d ). In addition, expression of cyclin D1 , which is suppressed by RAR [41] , was markedly lower in tumours of 16:0 fed mice ( Fig. 6d ). Notably, expression of the proliferation marker Ki67 was lower and apoptosis was more pronounced in tumours of 16:0 fed mice ( Fig. 6f ). Expression of the endoplasmic reticulum stress markers Chop and Grp78 were similar in tumours of mice fed the three diets ( Supplementary Fig. 6e ), indicating that the growth-inhibitory activity of 16:0 did not originate from initiation of endoplasmic reticulum stress. 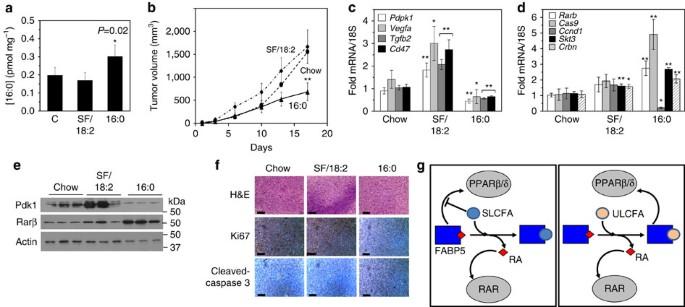Figure 6: 16:0 shifts RA signalling and suppresses mammary tumour growthin vivo. (a) Concentrations of 16:0 in tumours of mice fed denoted diets. Mean±s.d. (n=6). **P<0.01 by unpairedt-test versus chow control. (b) NaF cells (2 × 106) were transplanted into the mammary fat pad of NCr athymic female mice fed denoted diets and tumour growth was monitored. Mean±s.d. (n=6). **P<0.01 by unpairedt-test versus chow control. (c,d) mRNAs for PPARβ/δ (c) or RAR target genes (d) in mice fed denoted diets. Mean±s.d. (n=6). *P<0.05, **P<0.01 calculated by unpairedt-test. (e) Immunoblots demonstrating expression of PDPK1 and RARβ in tumours of mice fed denoted diets. Blots are representative data from 3 individual mice per group. (f) Immunohistochemistry analyses demonstrating expression of Ki67 and cleaved caspase 3 in tumours of mice fed denoted diets. Representative images out of three tumours per group are shown. Magnification 400 × , scale bars represent 50 μm. (g) A model illustrating the mechanism by which SLCFA and ULCFA regulate RA signalling. Left: SLCFA compete with RA and other PPARβ/δ ligands for binding FABP5, divert RA to RAR and inhibit PPARβ/δ activation. Right: ULCFA bind to FABP5 and divert RA to RAR. ULCFA are delivered to PPARβ/δ by FABP5 and activate it. Figure 6: 16:0 shifts RA signalling and suppresses mammary tumour growth in vivo . ( a ) Concentrations of 16:0 in tumours of mice fed denoted diets. Mean±s.d. ( n =6). ** P <0.01 by unpaired t -test versus chow control. ( b ) NaF cells (2 × 10 6 ) were transplanted into the mammary fat pad of NCr athymic female mice fed denoted diets and tumour growth was monitored. Mean±s.d. ( n =6). ** P <0.01 by unpaired t -test versus chow control. ( c , d ) mRNAs for PPARβ/δ ( c ) or RAR target genes (d) in mice fed denoted diets. Mean±s.d. ( n =6). * P <0.05, ** P <0.01 calculated by unpaired t -test. ( e ) Immunoblots demonstrating expression of PDPK1 and RARβ in tumours of mice fed denoted diets. Blots are representative data from 3 individual mice per group. ( f ) Immunohistochemistry analyses demonstrating expression of Ki67 and cleaved caspase 3 in tumours of mice fed denoted diets. Representative images out of three tumours per group are shown. Magnification 400 × , scale bars represent 50 μm. ( g ) A model illustrating the mechanism by which SLCFA and ULCFA regulate RA signalling. Left: SLCFA compete with RA and other PPARβ/δ ligands for binding FABP5, divert RA to RAR and inhibit PPARβ/δ activation. Right: ULCFA bind to FABP5 and divert RA to RAR. ULCFA are delivered to PPARβ/δ by FABP5 and activate it. Full size image These studies establish that RA activates both RAR and PPARβ/δ in vivo , and that the iLBP FABP5 is a critical regulator of both receptors. The observations further reveal that, through targeting FABP5, the important dietary components LCFA can regulate gene expression by governing the transcriptional activities of both RA-responsive nuclear receptors. We thus define a novel function for these fundamental biological building blocks. Taken together, the observations suggest the model depicted in Fig. 6g . SLCFA displace RA and other PPARβ/δ ligands from FABP5 and thereby block the delivery of such ligands to this receptor and inhibit its activation. Displacement of RA from FABP5 diverts the hormone to RAR, and as SLCFA do not induce either the nuclear import of FABP5 (ref. 32 ) or the transcriptional activity of PPARβ/δ (ref. 15 ), these LCFA concomitantly activate RAR and inhibit PPARβ/δ. On the other hand, binding of ULCFA to FABP5 similarly reroutes RA to RAR, but these compounds trigger translocation of FABP5 to the nucleus where they are delivered to PPARβ/δ and induce its activation. ULCFA thus activate both RAR and PPARβ/δ. Importantly, in vivo , LCFA shifted RA signalling when provided as dietary components, and, in cultured cells, they exerted such an effect at remarkably low concentrations. Hence, while SLCFA induce lipotoxicity and endoplasmic reticulum stress at concentrations of ∼ 500 μM (ref. 5 ), these compounds regulate the transcriptional activities of RAR and PPARβ/δ at <10 μM levels. Moreover, even in the absence of ectopic administration, short-term inhibition of fatty acid metabolism was sufficient to markedly induce expression of RAR target genes. The data thus show that the transcriptional activity of RAR is exquisitely sensitive to small alterations in cellular LCFA concentrations. Notably, while LCFA-induced activation of RAR critically depended on the presence of RA, PPARβ/δ was active and its activity was inhibited by 16:0 even in the absence of RA. These observations likely reflect that cells contain multiple endogenous ligands for PPARβ/δ and reveal that SLCFA suppress the activation of this receptor regardless of the nature of the agonist it uses under particular circumstances. The ability of LCFA to modulate gene expression by governing RA signalling is expected to have profound and wide-ranging consequences for cell function. One example addressed here is their involvement in regulating carcinoma cell growth. We show that, in FABP5-expressing carcinoma cells, SLCFA inhibit and ULCFA induce cell proliferation. We show further that, in such carcinomas, SLCFA convert RA from a pro-proliferative to a growth-inhibitory agent, induce apoptosis, suppress oncogenic properties and inhibit tumour development in vivo. SLCFA induced the expression of multiple RAR targets and reduce the levels of multiple PPARβ/δ target genes, many of which have a known function in cancer. Taken together with the reports that expression of FABP5 is upregulated and is associated with poor survival in several types of human cancers [22] , [23] , [24] , [26] , [28] , the data indicate that compounds that inhibit FABP5 may constitute a promising new class of drugs for therapy of certain types of cancer. While SLCFA function as potent FABP5 inhibitors, their rapid metabolism and potentially detrimental activities at pharmacological concentrations preclude their use as efficacious drugs. However, the data presented here provide precise criteria for developing FABP5 inhibitors and a strong proof-of-principle for the efficacy of such compounds in suppressing carcinoma cell growth. Reagents All-trans RA, 16:0, 18:0, 18:1 and 18:2, K 3 Fe(CN) 6 , K 4 Fe(CN) 6 . 3H 2 O and MgCl 2 were purchased from Sigma. GW1516 (GW), TTNPB and antagonists for RARα, RARβ and RARγ (BMS 195614, LE 135 and MM 11253, respectively) were purchased from Tocris Biosciences. The pan-RAR antagonist AGN193109 was purchased from Santa Cruz. The pan-RAR antagonist LE450 was a gift from Hiroyuki Kagechika (University of Tokyo). X-gal was from Fisher Scientific. The PPARβ/δ antagonist PT-S58 was synthesized using the protocol described in ref. 40 , 42 . Cells NaF, COS-7, MDA-MB-23, MCF-7 and HaCaT cells were cultured in DMEM supplemented with 10% fetal bovine serum (Invitrogen Life Sciences, Carlsbad, CA). PC3M cells were cultured in L -Glutamine-containing RPMI medium supplemented with 10% fetal calf serum (Invitrogen Life Sciences). HMEC cells were cultured in HMEC ready medium (Invitrogen Life Sciences). NaF cells were a gift from PhilipLeder (HarvardMedicalSchool, Boston, MA), HMEC cells were purchased from Thermo Fisher Scientific (A10565), COS-7, MDA-MB-23, MCF-7 and HaCaT cell lines were purchased from ATCC. For generation of NaF and HaCaT cell lines, lentiviral vectors pLKO.1-puro encoding respective short hairpin RNA targeting mouse and human FABP5, respectively, (Open Biosystems, AL, USA) were packaged in HEK293T cells by co-transfecting with pCMV and pMD2G. Virus was harvested 1–2 days after transfection and used to infect the cells. Single clones were selected using 10 μg ml −1 puromycin. MCF-7 cells were transfected with human FABP5 subcloned into pEGFP-N3 expression vector [32] using TransIT-BrCa reagent (Mirus Bio, LLC). The small interfering RNAs (Dharmacon) were transfected into NaF cells using Lipofectamine 2000 (Life Technologies). Endoplasmic reticulum stress assay For treatments with high 16:0 concentrations, the FA was complexed with bovine serum albumin (BSA). BSA (affymetrix) was delipidated using activated charcoal. 16:0 was dissolved in ethanol and added to the BSA solution to create a stock solution of 1 mM 16:0. The solution was incubated at 55 °C and for 30 min, then filtered and diluted in cell media to establish the desired concentrations. Mice PPRE–luc mice (RepTOP PPRE–Luc) [35] were obtained from Charles River laboratories. RARE–lacZ mice, which globally express β-galactosidase (lacZ) gene under the control of the RARE of the RA target gene Rarb [34] were purchased from Jackson Laboratories. FABP5 −/− mice [43] on a C57BL/6J background were provided by Gokhan Hotamisligil (Harvard School of Public Health). To generate the experimental groups RARE–LacZ +/− /FABP5 −/− ( n =6) and PPRE–luc +/− /FABP5 −/− ( n =6), each of the reporter lines was crossed with FABP5 −/− mice. For xenografts experiments, female NCr nude mice were obtained from the Athymic Animal and Xenograft Core Facility at the Case Western Cancer Center. All mice experiments were performed under the American Association for Accreditation of Laboratory Animal Care guidelines. All experimental protocols were approved by the Institutional Animal Care and Use Committee of Case Western Reserve University (protocol 2013-0040). Mice were maintained on a 12 h light and dark cycle and had access to water and diet ad libitum. Mouse experiments RARE–lacZ and PPRE–luc males and females (4–6 weeks old, n =3 each) were treated with RA (1 or 4 mg). PPRE–luc mice (4–6 weeks old, n =3) were used for GW (4 mg) treatments. Ligand solutions were prepared immediately before use in a vehicle of sterile saline:polyethylene glycol:Tween 80 (80:10:10 v/v) and injected intraperitoneally. For AGN193109 treatments, a total of six RARE–lacZ males were used (three mice treated and three controls). AGN193109 solution was prepared to a final concentration of 1 mg kg −1 and administered by intraperitoneal injections. Mice were treated with AGN193109 and then co-injected with RA the following day. RARE–lacZ and PPRE–luc males and females (4–6 weeks old, n =6), were used. Mice were fed ad libitum with a denoted diet and the reporter activity was measured a week later either by X-gal staining or imaging. At the end point, PPRE–luc mice were treated with RA, and imaged again 6 h later. Mouse diets (BioServ, Frenchtown, NJ) contained 18.1% protein, 4.8% fibre and 2.2% ash. Regular chow contained 7.1% fat, 59.3% carbohydrate and a total of 3.74 kcal g −1 (see http://www.bio-serv.com/pdf/F3156_F3197.pdf for composition). Diets enriched with palmitate or safflower oil contained 20.1% fat, 47.8% carbohydrate and a total of 4.4 kcal g −1 . Safflower-enriched diet contained 20% (g/g) safflower oil. Palmitate-enriched diet contained 17% palmitate (98%) and, to ensure adequate supply of essential fatty acids, 3% safflower oil. Nine-week-old NCr nude females were fed ad libitum and the amount of food consumed was recorded once a week. 1 week after being set on the diet, 2 × 10 6 NaF cells were injected subcutaneously into the mammary fat pad of the mice. Tumour size was assessed twice per week using a digital caliper. Tumour volumes were determined by measuring the length ( l ) and the width ( w ) of the tumour and calculating the volume ( V = lw 2 /2). Mice were scarified 23 days after injection. Statistical significance between the control and treated mice in both experiments was evaluated using a Student’s t -test. Mouse experiments were conducted after approval by the institutional animal care and use committee at Case Western Reserve University. Serum and tumours total free fatty acid concentrations were measured using the Serum/Plasma Fatty Acid Detection Kit (Zen-Bio). X-gal staining RARE–LacZ mice were killed and organs were harvested and fixed in 4% paraformaldehyde (1 h). Organs were washed three times with PBS, transferred into X-gal staining solution (20 mM K 3 Fe(CN) 6 , 20 mM K 4 Fe(CN) 6 .3H 2 O, 2 mM MgCl 2 , 1 mg ml −1 X-gal substrate) and incubated overnight at 37 °C. Organs were washed with PBS and imaged. In addition, fixed organs were embedded in paraffin, sectioned (8 μm), mounted on glass slides and counterstained with nuclear fast red before imaging. In vivo imaging PPRE–luc mice were injected intraperitoneally with luciferin (20 mg ml −1 , 200 μl) and imaged 5 min later by using IVIS 200 CCD camera (Xenogen, CA, USA). Immediately after, mice were killed and organs were harvested and imaged. Data acquisition and quantification were done with the software Living Image (Xenogen). MTT proliferation assays 1,000 cells were plated in quadruplicates in a 96-well plate and treated with ligand for 4 days. Cells were incubated with MTT reagent (5 mg ml −1 in PBS) until the formation of formazan crystals. Crystals were dissolved in 4 mM HCl in isopropanol, and absorbance at 590 nm was measured using a microplate reader. Transactivation assays COS-7 or HaCaT cells were cultured in six-well plates and co-transfected with either a luciferase reporter driven by three copies of a PPRE and expression vector for PPARβ/δ, or a luciferase reporter driven by RARE and expression vector for RARα, together with a vector harbouring cDNA for β-galactosidase, serving as a transfection control. 18 h post-transfection, cells were placed in a serum-free medium and treated with ligand. 18 h later, cells were lysed, luciferase activity was assayed (Promega, WI, USA) and corrected for transfection efficiency by the activity of β-galactosidase. Quantitative real-time PCR RNA was extracted using TRIZOL (Molecular Research Center). cDNA was generated using GeneAmp RNA PCR (Applied Biosystems). Quantitative real-time PCR was carried out using TaqMan chemistry and Assays-on-Demand probes (Applied Biosystems). The following probes were used: Caspase 9 Mm00516563_m1, Ccnd1 Mm00432359_m1, Cd47 Mm00495011_m1, Crbn Mm01182416_m1, Cyp26a1 Mm00514484_g1, Ddit3 (CHOP-10) Mm01135937_g1, Grp78 Mm00517690_g1, Pdpk1Mm00440707_m1, Plin2 Mm00475794_m1, Rarb Mm01319677_m1, Stk3 Mm00490480_m1, Tgfb2 Mm00436955_m1 and Vegfa Mm01281449_m1. 18s 4352930 (Applied Biosystems) ribosomal RNA was used for normalization. Relative expression was calculated as 2 −ΔΔCT for cell culture experiments and as 2 −ΔCT for tumours. Transcriptome analyses Two experiments were done: (1) NaF cells were cultured in media supplemented with 10% charcoal-treated FBS for 48 h and then treated with vehicle, GW (1 μM), RA (1 μM) or TTNPB (1 μM) for 6 h. (2) NaF cells were cultured in media supplemented with 10% FBS then treated with vehicle or 16:0 (10 μM) for 6 h. Total RNA was extracted by QIAzol (Qiagene) and purified using RNeasy columns (Qiagen). Samples were amplified, labelled, and hybridized on Affymetrix Mouse Gene 2.1 ST Arrays (Affymetrix, USA) by the Gene Expression and Genotyping Facility of the Case Comprehensive Cancer Center of Case Western Reserve University. Raw data files were analysed using Partek-Genomics-Suite (PGS) v6.6 software. Data was normalized using Robust Multichip Average Method, which allows reduction of block effect done at the probe-set level. T -test analysis was used to select differentially expressed genes with Fold Change and P -value cutoffs respectively fixed to at 1.2 and 0.05. Each treatment was compared with its relevant control. The network of genes with known functions in cancer was identified using Ingenuity Pathway Analysis (IPA) (Ingenuity Systems) ( P =2.2 × 10 −4 ). Immunoblots Total cell protein was extracted using RIPA buffer (25 mM Tris-HCl, 150 mM NaCl, 1% NP40, 1% sodium deoxycholate, 0.1% SDS). Proteins were resolved by electrophoresis on SDS–PAGE gels and transferred onto nitrocellulus membrane. Membranes were incubated with primary antibodies, followed by washes with Tween-TBS, and incubation with horse-radishperoxidase-conjugated antibodies. Protein expression was detected by exposure to enhanced chemiluminescence (ECL) and exposed to XR-B X-ray film. Band intensities were quantified using ImageJ 1.40 g software (Wayen Rasband, NIH, USA). Antibodies against Cleaved caspase 3 (9661) and PARP (9532) were purchased from Cell Signaling. Antibodies against Actin (sc-47778), Caspase 9 (sc-7885), RARb (sc-7179) and Tubulin (sc-9104) were purchased from Santa Cruz Biotechnology. Antibodies against FABP5 and PDPK1 were purchased form R&D Systems (AF1476 and AF3077, respectively) and BD Transduction Laboratories (611070), respectively. All antibodies were used at 1:1,000 dilution. Uncropped scans of western blots shown in Figs 4g,j,m and 6e are presented in Supplementary Fig. 7 . Colony formation assays A layer of 0.8% agarose in cell media was cast in a six-well plate and set in room temperature to solidify. Cells were suspended in 0.25% agarose in media and 1 ml from this mixture containing 5,000 cells was added to each well. Cells were cultured for 21 days. Media were replenished every 3 days. Colonies were visualized by staining with 0.005% crystal violet and counted under a light microscope. Palmitic acid analysis Palmitic acid was quantified using stable isotope dilution liquid chromatography with on-line tandem mass spectrometry using a modification of a method previously described (1). For serum samples, palmitic acid-7,7,8,8-d 4 internal standard (DLM-2893, Cambridge Isotope Laboratories, Inc.) was added to serum before acidification with acetic acid, and the palmitic acid was extracted into hexane [44] . For tumour tissues, samples were homogenized in methanol, and to an aliquot, palmitic acid-7,7,8,8-d 4 added as internal standard. Samples were then acidified and extracted with hexane as with serum samples. For all analyses hexane extracts were dried under N 2 , resuspended in methanol, and injected onto a reverse phase C18 HPLC column (2.0 × 150 mm, 5 μm, Phenomenx, Torrance, CA) operated at a flow rate of 0.2 ml min −1 and resolved using a linear gradient between 0.2% formic acid in water and 0.2% formic acid in acetonitrile. HPLC column effluent was introduced into an AB Sciex API 5000 triple quadrupole mass spectrometer using electrospray ionization in negative-ion mode. Analytes were monitored using multiple reaction monitoring of parent and characteristic daughter ions: m/z 255 → 237 for palmitic acid; and m/z 259 → 241 for palmitic acid-7,7,8,8-d 4 . Immunohistochemistry Antigen retrieval was done by boiling the slides in 10 mM citric buffer (pH 6.0, 15 min). Apoptosis and cell proliferation were examined by immunohistochemical analyses using rabbit polyclonal antibody recognizing cleaved caspase 3 (Cell Signaling, no. 9661; dilution 1:200), and Ki67 (Novocastra Laboratories, no. NCL-Ki67p; dilution 1:500), respectively. Primary antibodies were incubated with deparaffinized sections (overnight at 4 °C). Sections were incubated (30 min) with biotinylated secondary antibody and detected with EnVision System-HRP (DAB) (Dako) kit. Binding assays Assays were carried out by fluorescence titrations. FABP5 was bacterially expressed and purified and the equilibrium dissociation constants (Kd) that characterize its interactions with different FAs were measured by fluorescence competition assays. The method entails two steps [37] . In the first step, Kd for the association of the protein with the fluorescent fatty acid probe ANS was measured. Protein (1 μM) was titrated with ANS from a concentrated solution in ethanol. Ligand binding was monitored by following the increase in the fluorescence of the ligand on binding to the protein, and Kd for the association of ANS with FABP5 was computed from titration curves [45] . Kds for binding of non-fluorescent ligands were then measured by monitoring their ability to compete with ANS for binding to the protein. FABP5 was pre-complexed with ANS at 1:1 molar ratio and titrated with the different FAs whose binding was reflected by a decrease in probe fluorescence. Kds were extracted from the EC50 of the competition curve and the measured Kd for ANS. Analyses were carried out using Origin 8 software (MicroCal Software, Inc., Northampton, MA). Statistics Statistical significance was analysed using an independent sample t -test versus respective untreated controls. Accession codes. The microarray data have been deposited in the NCBI Gene Expression Omnibus (GEO) database under accession code GSE73186 . How to cite this article: Levi, L. et al . Saturated fatty acids regulate retinoic acid signalling and suppress tumorigenesis by targeting fatty acid-binding protein 5. Nat. Commun. 6:8794 doi: 10.1038/ncomms9794 (2015).